Giant Rashba splitting in graphene due to hybridization with gold Graphene in spintronics is predominantly considered for spin current leads of high performance due to weak intrinsic spin–orbit coupling of the graphene π electrons. Externally induced large spin–orbit coupling opens the possibility of using graphene in active elements of spintronic devices such as the Das-Datta spin field-effect transistor. Here we show that Au intercalation at the graphene–Ni interface creates a giant spin–orbit splitting (~100 meV) of the graphene Dirac cone up to the Fermi energy. Photoelectron spectroscopy reveals the hybridization with Au 5 d states as the source for this giant splitting. An ab initio model of the system shows a Rashba-split spectrum around the Dirac point of graphene. A sharp graphene–Au interface at the equilibrium distance accounts for only ~10 meV spin–orbit splitting and enhancement is due to the Au atoms in the hollow position that get closer to graphene and do not break the sublattice symmetry. Graphene shows fascinating electronic properties because of its structure consisting of two equivalent sublattices A and B that determine its band structure with the linear dispersion near conical and points in reciprocal space. A and B are identified as a pseudospin, and the isospin indicating and valleys is a conserved quantum number. In addition to the pseudo- and isospin, the real spin is of critical importance for the properties of graphene [1] , [2] , [3] , [4] , [5] , [6] , [7] , [8] , [9] , [10] , [11] , [12] . The intrinsic spin–orbit coupling in graphene is very weak [3] , [4] , [5] . The main contribution to it originates from the coupling to the graphene d orbitals [9] . The resulting splitting is of the order of only 0.05 meV [10] , which, together with the high carrier mobilities, suggests a long spin-coherence length. The measured values reach 1.5–2 μm [3] , [4] , [5] , whereas the theoretical predictions are even by an order of magnitude higher. Hence, it is at present unclear whether these values represent the practical limits [7] . We have recently measured the spin–orbit splitting in graphene of Δ so =13 meV [12] . This splitting occurs in the graphene/Ni(111) system after a Au monolayer is intercalated by heating between the graphene and the Ni substrate [13] . This Au layer serves a dual purpose: on the one hand, it transforms the graphene monolayer from the one strongly bonded to Ni(111) [14] into a quasifreestanding one. This decoupling effect is apparent from the resulting linear quasirelativistic π bands of the graphene, that is, the Dirac cone [12] , [15] , [16] . On the other hand, the Au interlayer produces a different type of the spin–orbit splitting, which is extrinsic. Indeed, the spin–orbit coupling is known to be important at the surface of Au [17] and in Au nanowires [18] , and Au(111) is frequently considered as a model for the Rashba effect induced by breaking the up-down symmetry [17] , [19] . A large Rashba effect on graphene would open the possibility of using this material in active elements of spintronic devices such as the Das-Datta spin field-effect transistor [6] , [11] . For graphene with its two-atom basis (sublattices A and B) and additionally broken up-down symmetry, the band dispersion including the spin–orbit coupling has been calculated in a recent work [20] , where the dependence of spin polarization on the two-dimensional electron wave vector k || was also found. In a zero magnetic field, the band topology was predicted to be similar to that of the unbiased spinless bilayer graphene but with an additional spin texture, which is tangential to the circular constant-energy surfaces. Spin and pseudospin are coupled in such a way that the contributions from both A and B sublattices lead to a substantial spin interference in the photoemission process [21] . Here we show by means of spin- and angle-resolved photoelectron spectroscopy that an extrinsic spin–orbit splitting Δ s o of the order of 100 meV can be obtained in graphene near the Fermi energy, which is an enhancement by an order of magnitude relative to our previous finding [12] . We reveal different types of the superstructures characteristic to the graphene–Au interface and determine the spin-dependent hybridization, which changes with the evolution of superstructure geometry. Based on our ab initio calculations, the giant spin–orbit splitting is attributed to dilute Au atoms that are in a closer vicinity of the carbon atoms than the Au monolayer. Giant spin splitting of Dirac fermions in graphene Fig. 1 shows the spin- and angle-resolved photoemission measurements of graphene/Au/Ni(111). Fig. 1a shows the π band with its linear quasirelativistic dispersion, and crosses indicate where spin-resolved photoemission spectra ( Fig. 1b–e ) have been measured. The splitting between spin-up spectra I ↑ ( E ) (upward triangles) and spin-down spectra I ↓ ( E ) (downward triangles) is clearly visible, and amounts to 90 meV at k || =1.65 Å −1 and −105 meV at k || =−1.65 Å −1 . Apparently, the sign of the splitting reverses with the sign of k || as expected for a Rashba effect ( Fig. 1d ). This giant spin splitting constitutes our central experimental result. The splitting exceeds also the room-temperature broadening, and together with the fact that it extends to the Fermi energy, this makes it directly relevant for transport applications. In fact, transport properties of graphene with an externally induced spin–orbit splitting have been intensively investigated in recent years [22] , [23] , [24] , and important predictions have been made: the spin Hall effect [22] , the quantum spin Hall effect [2] , [23] and, with an additional exchange interaction, the quantum anomalous Hall effect [24] . 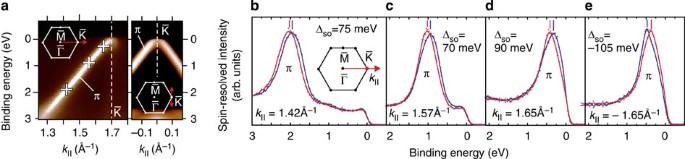Figure 1: Giant spin–orbit splitting Δsoof the graphene π band. (a) Angle-resolved photoemission near thepoint of the graphene Brillouin zone of graphene/Au/Ni(111). Crosses indicate where the Dirac cone of the graphene π-states is probed by (b–e) spin- and angle-resolved photoemission spectra (hν=62 eV). Blue and red lines at panels (b–e) are spin-up and spin-down spectra.k||is an in-plane component of the wave vector. The spin splitting reverses with the sign ofk||. At panels (a,b), the directions in the graphene Brillouin zone where corresponding measurements were done are shown in insets. Figure 1: Giant spin–orbit splitting Δ s o of the graphene π band. ( a ) Angle-resolved photoemission near the point of the graphene Brillouin zone of graphene/Au/Ni(111). Crosses indicate where the Dirac cone of the graphene π-states is probed by ( b – e ) spin- and angle-resolved photoemission spectra ( hν =62 eV). Blue and red lines at panels ( b – e ) are spin-up and spin-down spectra. k || is an in-plane component of the wave vector. The spin splitting reverses with the sign of k || . At panels ( a , b ), the directions in the graphene Brillouin zone where corresponding measurements were done are shown in insets. Full size image To establish the connection between our previous 13 meV data and the new 100 meV data, we undertook a closer inspection of the spin-resolved spectra of Fig. 1 . They reveal that the system is inhomogeneous and the high-splitting phase (~100 meV) and the low-splitting phase (~10 meV) are present simultaneously. Line fits and spectral decompositions ( Supplementary Fig. S1 ) show that the high-splitting phase makes up between one-third and two-thirds of the spectral weight, corresponding, roughly speaking, to a half of the sample region of about 200 × 200 μm 2 that is probed simultaneously. The decomposition is possible because of an energy shift between the two phases, with the low-splitting phase observed at about 200–500 meV higher binding energy. The giant magnitude of the splitting and the distribution of the spectral weight between the high-splitting and low-splitting phases ranging from 1:2 to 2:1 have been reproduced in several in situ preparations and at different beamlines. Hybridization with Au 5 d states as the source of giant splitting We want to unveil the electronic origin of this strongly enhanced spin splitting including the reason for its nonuniformity and the relation to our previous results. Direct probing as well as controlling of the Au interlayer that is the likely source of the giant Rashba splitting are challenging because most of the Au atoms are located underneath the graphene layer. Basically, we can only control the nominal amount of Au deposited on top of the graphene/Ni before intercalation, which typically exceeds the subsequently intercalated amount. Although graphene and Ni(111) have a lattice mismatch of only 1.2%, the mismatch between the graphene and Au(111) is much larger (~14%). Therefore, the intercalated monolayer of Au cannot reach the same atomic density as the Ni. Probing of the resulting interfacial structure is possible by scanning tunnelling microscopy (STM) ( Fig. 2a ) and by low-energy electron diffraction (LEED) ( Fig. 2b ). Indeed, the moiré effect reveals the superstructure through the periodic beating developing because of the mismatch between the graphene lattice and the Au monolayer. Moreover, the photoemission signal from the Au 5 d states under the graphene is very well visible. 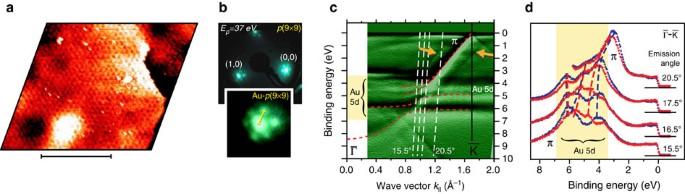Figure 2: Geometrical structure and hybridization of the Au monolayer under graphene. (a) STM and (b) LEED for 1.1 monolayer (ML) of gold under the graphene layer with a 9 × 9 moiré-type superstructure. A scale bar at the panelacorresponds to 400 Å. (c) Angle-resolved photoemission (first derivative of the intensity over energy). Hybridization between π state of graphene and 5dstates of Au is emphasized by the dashed red lines. Orange arrows show π-band replicas shifted to the larger and smallerk||values because of the 9 × 9 superstructure. White dashed lines denote thek||values for which the spin-resolved spectra displayed indwere measured (hν=62 eV). (d) Spin-resolved measurements in the region of hybridization between the graphene and gold bands. It is seen that the spin–split π states develop directly out of a large spin–orbit splitting of Au 5dstates. Blue and red triangles denote spectra for opposite spin. Blue and red dashed lines emphasize dispersion of bands. Yellow-shaded area shows the region of Au 5dstates. Figure 2: Geometrical structure and hybridization of the Au monolayer under graphene. ( a ) STM and ( b ) LEED for 1.1 monolayer (ML) of gold under the graphene layer with a 9 × 9 moiré-type superstructure. A scale bar at the panel a corresponds to 400 Å. ( c ) Angle-resolved photoemission (first derivative of the intensity over energy). Hybridization between π state of graphene and 5 d states of Au is emphasized by the dashed red lines. Orange arrows show π-band replicas shifted to the larger and smaller k || values because of the 9 × 9 superstructure. White dashed lines denote the k || values for which the spin-resolved spectra displayed in d were measured ( hν =62 eV). ( d ) Spin-resolved measurements in the region of hybridization between the graphene and gold bands. It is seen that the spin–split π states develop directly out of a large spin–orbit splitting of Au 5 d states. Blue and red triangles denote spectra for opposite spin. Blue and red dashed lines emphasize dispersion of bands. Yellow-shaded area shows the region of Au 5 d states. Full size image On the contrary, the core levels do not allow to draw any conclusions about the structure of gold under the graphene layer as the shape and the energy positions of the 4 f states of Au do not change during the intercalation process. This is shown, as an example, for graphene on Co(0001) in the Supplementary Fig. S2 . For observing the spin–orbit splitting of the size of 100 meV in the graphene/Au system, spin-resolved ARPES (angle-resolved photoemission spectroscopy) measurements are required because the ARPES spectrum without the spin resolution reveals only a sharp peak without any apparent splitting ( Supplementary Fig. S3 ). Figures 1a and 2c show that the graphene electronic structure resembles that of the freestanding graphene. The Au layer prevents any conceiveble carbon–Ni hybridization. Nevertheless, also in the quasifreestanding phase with intact Dirac cone ( Fig. 2c ), several hybridization points between the π states of graphene and 5 d states of Au are revealed at the binding energies between 4 and 6.5 eV. In addition, replicas of the graphene π-band shifted to smaller and larger values of the wave vector k || are observed (orange arrows in Fig. 2c ). Their shift in k || amounts to between 1/7 and 1/9 of the distance. The STM image in Fig. 2a shows a moiré pattern of a similar periodicity. The observed superstructure can be identified by the LEED more accurately as a 9 × 9 ( Fig. 2b ). This is in a good agreement with the periodicity of the band replicas in the photoemission spectra. Dashed lines in Fig. 2c show where we probed the hybridization points by the spin-resolved spectra ( Fig. 2d ). These spectra reveal that the giant ~100 meV spin splitting of the π-band smoothly merges into an even larger spin splitting (~0.6 eV) of the Au 5 d states. This provides a strong indication that the spin-dependent hybridization of the carbon π states with the d states of the heavy Au is the origin of the giant Rashba splitting in graphene. For probing similar spin-polarized spectra of the gold states, spin-resolved measurements for two opposite directions of the in-plane wave vector were performed, and the results are shown in the Supplementary Fig. S4 . Interestingly, when a larger nominal amount of Au is deposited on top of graphene before intercalation, after intercalation it forms a slightly different 8 × 8 superstructure. Supplementary Figures S5 and S6 show the characterization by STM, LEED and ARPES of the graphene/Au/Ni(111) systems intercalated by a different amount of Au in which the 9 × 9 and 8 × 8 superstructures manifest themselves. An extra hybridization of the graphene π-band and the Au d states around the 3 eV binding energy is typical of the 8 × 8 superstructure. However, this hybridization does not further enhance the giant spin–orbit splitting ( Supplementary Fig. S7 ), which indicates that the differences between the 9 × 9 and 8 × 8 superstructures have no role in the giant spin–orbit splitting. In addition to the graphene/Au/Ni system, the spectra from control samples characterized by absence of a detectable spin–orbit splitting were measured (graphene/SiC, Supplementary Fig. S8 and graphene/Cu, Supplementary Fig. S9 ). Theory Now, we turn to ab initio theory to clarify the origin of the giant spin splitting. Modelling the 9 × 9 or 8 × 8 superstructures of the graphene/Au/Ni system, which would increase the unit cell by two orders of magnitude as compared with graphene, is unnecessary because both superstructures show a similar spin–orbit splitting. A p (1 × 1) structure with an on-top position for graphene on the Au monolayer has been chosen instead ( Fig. 3a ). 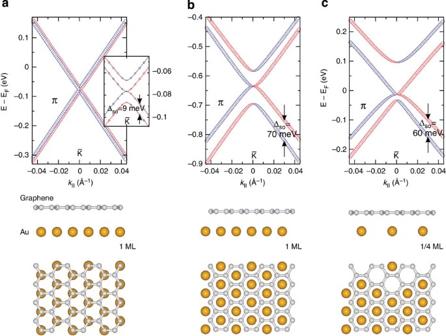Figure 3: Interface geometry and Dirac-cone splitting. (a) Results ofab initiocalculations showing the 9 meV Rashba-split Dirac cone for graphene on gold monolayer in the on-top position (open circles) at the equilibrium distance of 3.3 Å. In the inset, a magnified view near the Dirac point is shown; lines depict the dispersion as predicted from the analytical model20. (b) The Au monolayer is laterally moved to the graphene hollow sites and can now be pressed into the graphene to the non-equilibrium distance of 2.5 Å without breaking the Dirac cone but enhancing the spin–orbit splitting to 70 meV. (c) Improved model with the Au atoms still sitting in the graphene hollow sites but diluted to 0.25 ML Au in ap(2 × 2) geometry and at the equilibrium distance of 2.3 Å. Here a spin–orbit splitting of ~50–100 meV and intact Dirac cone are achieved. Blue and red lines at panelsa–cdenote spin-up and spin-down bands. Atomic structures are schematically shown at the bottom of each panel. Figure 3: Interface geometry and Dirac-cone splitting. ( a ) Results of ab initio calculations showing the 9 meV Rashba-split Dirac cone for graphene on gold monolayer in the on-top position (open circles) at the equilibrium distance of 3.3 Å. In the inset, a magnified view near the Dirac point is shown; lines depict the dispersion as predicted from the analytical model [20] . ( b ) The Au monolayer is laterally moved to the graphene hollow sites and can now be pressed into the graphene to the non-equilibrium distance of 2.5 Å without breaking the Dirac cone but enhancing the spin–orbit splitting to 70 meV. ( c ) Improved model with the Au atoms still sitting in the graphene hollow sites but diluted to 0.25 ML Au in a p (2 × 2) geometry and at the equilibrium distance of 2.3 Å. Here a spin–orbit splitting of ~50–100 meV and intact Dirac cone are achieved. Blue and red lines at panels a – c denote spin-up and spin-down bands. Atomic structures are schematically shown at the bottom of each panel. Full size image The distance between graphene and the Au ML is a parameter of an enormous influence on the spin–orbit splitting in graphene ( Supplementary Fig. S10 ). The fact that also the electron Fermi energy varies essentially with this distance allows us to make connection to the experiment. The experimental Fermi level corresponds with its slight p -doping (hole doping) to the distance 3.3–3.4 Å in the theoretical model, and data for the distance of 3.3 Å is shown in Fig. 3a . This is also the equilibrium distance calculated before for graphene/Au(111) [25] . According to analytical prediction, the band topology is peculiar around the point with two pairs of bands—a gapped one and a non-gapped one [20] , [21] . This analytical model [20] , [21] does not assume any specific surface configuration. The bands have so far been confirmed for freestanding graphene in a supercell geometry by density functional theory calculations for an applied field E =4.0 V nm −1 [9] (ref. 9 ) and for the field E realistically created by the interface to Au giving a spin–orbit splitting of 8 meV [26] . This was done in Fig. 3a that shows the spin–orbit split bands at the Dirac point at for the on-top geometry. In the inset, these ab initio results (symbols) are magnified near the Dirac point and compared with the dispersion of the analytical model (solid line), which is fully confirmed. This is also important for the predicted magnetic-field dependence [20] . In agreement with the experiment, our ab initio calculation reveals C π-Au d hybridization as the source of the spin–orbit splitting in the graphene. The graphene π-band ( p z orbitals) hybridizes indeed with the deeper Au 5 d bands of and d yz type because of their matching symmetry. Despite the large distance of 3.3 Å the hybridization is strong, which has not been considered in the literature in connection with graphene–noble–metal interfaces. This is best seen after the spin–orbit coupling is turned off leaving only gaps caused by hybridization: we determine hybridization gaps of widths and E g , yz ≈0.5 eV ( Supplementary Fig. S11 ). Their absolute binding energies do not compare well with the experiment revealing the limitations of the Au monolayer as model substrate. This situation improves largely and the main C π-Au d hybridization moves from ~3 to ~4 eV below E F when the Ni substrate is included in the calculation ( Supplementary Fig. S12 ). The spin–orbit splitting in Fig. 3a is 9 meV near E F but increases strongly when the distance between graphene and Au is reduced (see Supplementary Fig. S10 for the detailed dependence on the distance). On the other hand, the Dirac cone is destroyed at closer graphene–Au distance, giving, for example, for 2.5 Å a band gap of 40 meV at . The reason for this is the broken A-B symmetry of carbon atoms in the on-top geometry ( Fig. 3a ), which, remarkably, does not manifest itself very much at larger distances. On the contrary, a hollow-site geometry preserves the A-B symmetry in the graphene (see Fig. 3b ). Consequently, an intact Dirac cone is obtained in the hollow-site geometry also for smaller graphene–Au distances such as 2.5 Å in Fig. 3b . We are very well able to obtain at this arbitrary interlayer distance of 2.5 Å a giant spin–orbit splitting of ~70 meV. However, at such a close distance repulsive interactions cost as much as 1 eV relative to the equilibrium separation and this geometry is thus considered unrealistic. Although the giant spin–orbit splitting apparently is difficult to reproduce by density functional theory in equilibrium, the intact Dirac cone is not. The intact Dirac cone is presently obtained with p (1 × 1) on-top graphene/Au and has also been found for p (1 × 1) graphene/Cu(111) where the on-top position is determined to be energetically favourable [25] . Relative to this p (1 × 1) on-top geometry that implies maximum A-B symmetry breaking, a moiré superstructure such as the 9 × 9 one necessarily breaks the A-B symmetry to a lesser or vanishing degree, which is favourable for obtaining an intact Dirac cone. After having investigated other laterally shifted positions of the p (1 × 1) overlayer and a 4 × 3 moiré superstructure as well as corrugation in the graphene, all yielding spin–orbit splittings of the order of 10 meV at equilibrium graphene–Au distances, the conclusion is that the giant spin–orbit splitting will not be accounted for by the sharp graphene–Au interface alone that our structural characterization by LEED and STM suggests as simplest case. This means that a model for a realistic splitting will have to include individual Au atoms, which then can obtain a higher coordination to the carbon. Because of the resulting attraction and shorter distance, this allows for a stronger spin–orbit splitting on the graphene π-states. As seen above, at small graphene–Au separations, the preservation of A-B symmetry becomes critical and leads us once again to the hollow-site geometry. Figure 3c shows this situation for graphene/0.25 ML Au in a p (2 × 2) structure with the Au in the hollow site relative to the graphene. The distance between Au atoms and graphene layer is 2.3 Å (as for the Au monolayer of Fig. 3b ), which is the equilibrium distance determined by our structural optimization. Fig. 3c shows that this structure enhances the spin–orbit splitting to values between 50 and 100 meV while keeping the characteristic band topology and the Dirac point. This demonstrates that our experimental results are quite reasonable from the ab initio point of view. The 9 × 9 and 8 × 8 structures will include in the simplest case a substantial amount of Au atoms arranged in the hollow sites of graphene [27] but this does not imply a reduced distance, especially if one considers that 9 × 9 is also the structure, which a Au monolayer alone forms on Ni(111) [28] . Therefore, the 9 × 9 and 8 × 8 superstructures are probably not relevant for the giant splitting and both give rise to only ~10 meV splitting. The previously measured data [12] were characterized by a smaller ~13 meV spin–orbit splitting, and this low-splitting phase is in principle in agreement with our present calculations for the full Au monolayer. The published [12] band dispersion measured along reflects the presence of a sample with structural defects. It contained substantial contributions of rotated domains visible as characteristic dispersions, appearing along ( Supplementary Fig. S13 ), which is not the case in the present data even when the amount of intercalated Au is varied systematically from zero to >1 ML ( Supplementary Fig. S5 ). The intercalation process under the graphene, including that of Au, is at present far from understood. The accepted main route is via defects in the graphene [29] , and for large molecules this can be confirmed by STM directly [30] . The presence of many domain boundaries facilitates the intercalation and apparently results in the low-splitting phase. Intercalation of Au works, however, also in samples that are free of defects over large distances. The temperature of intercalation and that of the initial graphene formation are very similar in the graphene/Au/Ni(111) system so that an opening and closing of the graphene bonds seems possible during intercalation. This could lead to more Au atoms that are locally closer to the graphene, either as subsurface Au or as adatoms. The p (2 × 2) plot of Fig. 3c is useful for demonstrating that an enhancement of the spin–orbit coupling in graphene by sparsely distributed Au atoms is possible in an equilibrium structure, but it does not imply that the Au arrangement possesses such an ordered structure. We can exclude the substitution of carbon atoms by Au atoms. Their size would correspond to two carbon atoms, and the resulting distortion would manifest itself in STM. Another possibility are non-intercalated residual atoms above the graphene for which we have no direct experimental evidence. We mention that such atoms cannot be detected by our STM technique because they should be highly mobile on graphene and shifted along by the STM tip. To explore a realistic model that includes the Ni substrate, the band dispersion for a structure of graphene sandwiched between 0.25 and 1 ML Au on top of 3 ML Ni has been calculated as well ( Supplementary Fig. S14 ) and gives practically the same Dirac cone with giant spin splitting as in Fig. 3c . In summary, we report a giant Rashba splitting in graphene in contact with Au reaching up to 100 meV. This splitting is caused by graphene–Au hybridization. Although a flat Au monolayer can account for only ~10 meV spin–orbit splitting as has been reported previously [12] , a structure of laterally more separated Au adatoms residing in hollow-site positions closer to graphene provides at the equilibrium graphene–Au distance an enhanced spin splitting of Δ SO ~50–100 meV, a realistic Fermi-level position and an intact Dirac cone. We attribute simultaneous presence of both 100 and 10 meV splittings to the coexistence of areas with and without extra Au either as adatoms or immersed under the graphene. Experiments Angle-resolved photoemission spectra have been measured with a hemispherical analyser operated in parallel angular detection mode using a six-axes automated cryomanipulator. Spin- and angle-resolved photoemission has been performed with a hemispherical analyser coupled to a Rice University Mott-type spin polarimeter operated at 26 kV sensitive to the in-plane spin components perpendicular to k || . Linearly polarized synchrotron light from the UE112-PGM undulator beamlines at BESSY II has been used for excitation. Overall energy (of electrons and photons) and angular resolution of the experiments was 80 meV and 1° with both angle and spin resolution, and 6 meV and 0.3° with angle resolution only. The unmagnetized Ni(111) surface was prepared as a 15–20 ML thick film on W(110), and graphene was synthesized by cracking of propene at the Ni(111) surface held at T ~800 K. Because the surface reactivity drops drastically with the formation of graphene, this procedure results in exactly one graphene monolayer [14] . Intercalation of Au [13] was achieved by deposition of a nominal monolayer coverage of Au on the graphene followed by brief annealing at 750 K. This Au coverage was systematically varied in a wedge-type experiment. STM measurements were performed at room temperature using polycrystalline W tips carefully cleaned in situ . All experiments were done in ultra-high vacuum with a base pressure below 2 × 10 −10 mbar. Theory The calculations have been conducted in the generalized gradient approximation [31] to density functional theory, using the full-potential linearized augmented plane-wave method implemented in the FLEUR code ( http://www.flapw.de ). We use a plane-wave cutoff of 7.37 Å −1 and muffin-tin radii of 0.68 Å for carbon, 1.22 Å for Au and 1.16 Å for Ni. For the integration in reciprocal space, for example for the calculation of Fig. 3a , 49 k || points have been used in the two-dimensional Brillouin zone. Spin–orbit interaction is treated self-consistently as described by Li et al [32] . For simplicity, the Au monolayer was assumed to be pseudomorphic ( p (1 × 1)) to the graphene (graphene lattice constant 2.489 Å) and to the Ni(111) substrate with the same area density of Ni(111). This is also the basis for the 0.25 ML Au in the p (2 × 2) structure. The important Au–graphene distance has been chosen in Fig. 3a based on the Fermi-level position and in agreement with Giovannetti et al [25] as 3.3 Å. The dependence of the Fermi level and spin–orbit splitting on this parameter is shown in Supplementary Fig. S10 . For the calculation shown in Fig. 3c , a structural optimization has been conducted by force minimization. How to cite this article: Marchenko, D. et al. Giant Rashba splitting in graphene due to hybridization with gold. Nat. Commun. 3:1232 doi: 10.1038/ncomms2227 (2012).